Discordant timing between antennae disrupts sun compass orientation in migratory monarch butterflies To navigate during their long-distance migration, monarch butterflies ( Danaus plexippus ) use a time-compensated sun compass. The sun compass timing elements reside in light-entrained circadian clocks in the antennae. Here we show that either antenna is sufficient for proper time compensation. However, migrants with either antenna painted black (to block light entrainment) and the other painted clear (to permit light entrainment) display disoriented group flight. Remarkably, when the black-painted antenna is removed, re-flown migrants with a single, clear-painted antenna exhibit proper orientation behaviour. Molecular correlates of clock function reveal that period and timeless expression is highly rhythmic in brains and clear-painted antennae, while rhythmic clock gene expression is disrupted in black-painted antennae. Our work shows that clock outputs from each antenna are processed and integrated together in the monarch time-compensated sun compass circuit. This dual timing system is a novel example of the regulation of a brain-driven behaviour by paired organs. Each fall, millions of monarch butterflies ( Danaus plexippus ) from eastern North America undertake a breathtaking, long-distance migration to their overwintering grounds in central Mexico [1] , [2] , [3] . Monarchs use a time-compensated sun compass to orient in a southerly direction during the migration. The circadian clock provides the timing mechanism that allows for the adjustment of flight orientation to maintain a southerly bearing, even though the skylight cues used for directionality (for example, the azimuthal position of the sun) move across the sky during the day [4] , [5] , [6] . Previous work has shown that the time-compensated sun compass mechanism in migrating monarchs requires the antennae [7] . The antennae possess circadian clocks that provide the necessary timing component for accurate sun compass orientation. For example, migrants in which both antennae have been removed and thereby lack antennal clocks have disoriented group flight direction in flight simulator trials; they are no longer oriented in the southerly direction as found with intact fall migrants [7] . Similarly, migrants in which both antennae are painted black to block light input and thereby light entrainment of antennal clocks exhibit group flight orientation that differs substantially from non-manipulated monarchs [7] . Consistent with these results, the temporal patterns of clock gene expression in the antennae reveal that light-entrainable circadian clocks reside in these structures and that these clocks are no longer entrained by light when the antennae are painted black [7] . Even though the antennae are necessary for proper sun compass orientation in migratory monarchs, the relationship between each of the two antennae for accurate timing of the sun compass is unknown. We now report that one intact antenna (either the right or left) is sufficient for proper sun compass orientation. Surprisingly, rendering either antenna light insensitive by painting it black, while leaving the other light sensitive, disrupts sun compass orientation, whereas removing the black-painted antenna restores oriented flight. The patterns of circadian clock gene oscillations in the antenna and brain confirm the behavioural findings of disrupted sun compass orientation with competing timing signals from the two antennae. Thus, although the timing of the circadian clocks between the two antennae is not strongly coupled, time-encoding outputs from each antenna are ultimately integrated together in the monarch time-compensated sun compass circuit in the brain. One antenna is sufficient for sun compass orientation We first examined whether the right or left antenna is sufficient for fall migrants to orient in the southerly direction. Antennal laterality has been shown for olfactory learning in bees [8] , [9] , [10] and may also occur in relationship to the timing output between the right and left antenna of migratory monarchs. Flight simulator trials were performed on migrating monarchs with one antenna removed and housed indoors in either a 12-h light:12-h dark (LD) cycle, which was timed to coincide with the prevailing fall lighting cycle, or a 6-h-delayed LD cycle. The mean orientation vector ( α ) of migrants with a single left antenna housed in LD was 229.4° ( n =6, r =0.788, P =0.017, Rayleigh's test) ( Fig. 1a , red dots), while the α of those with a single right antenna was 206.8° ( n =6, r =0.932, P =0.001, Rayleigh's test) ( Fig. 1a , blue dots). The mean flight orientation of both migrant groups did not differ ( F 1, 10 =1.32, P =0.28, Watson–Williams F -test) and the combined α of both groups was 217.2° ( n =12, r =0.844, P <0.001, Rayleigh's test) ( Fig. 1a ). This southwesterly orientation direction is similar to that previously reported for the bulk of fall migrants housed in LD with both antennae intact [4] , [5] , [7] , [11] . 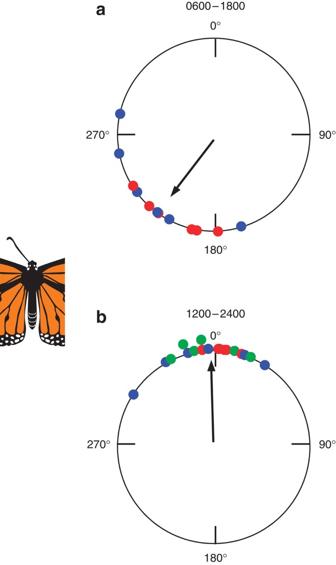Figure 1: A single antenna is sufficient for proper time-compensated sun compass orientation. (a) Flight orientation of migrants with only a single antenna and housed in LD (lights on between 0600 and 1800 hours EST). Migrants were flown between 1300 and 1500 hours from 29 September to 23 October 2010. The large circle represents the 360° of possible directions with 0°=north. The small solid circles on the perimeter represent the flight orientation of individual butterflies with blue dots representing those with a right antenna and red dots those with a left antenna. Arrow indicates the mean vector and the length of this arrow represents itsrvalue. Left, experimental condition of a generic monarch for (a) and (b). (b) Flight orientation of migrants with only a single antenna and housed in a 6-h-delayed LD cycle (light on between 1200 and 2400 hours). Migrants with both antennae intact were also tested in the 6-h-delayed LD cycle (green dots). Figure 1: A single antenna is sufficient for proper time-compensated sun compass orientation. ( a ) Flight orientation of migrants with only a single antenna and housed in LD (lights on between 0600 and 1800 hours EST). Migrants were flown between 1300 and 1500 hours from 29 September to 23 October 2010. The large circle represents the 360° of possible directions with 0°=north. The small solid circles on the perimeter represent the flight orientation of individual butterflies with blue dots representing those with a right antenna and red dots those with a left antenna. Arrow indicates the mean vector and the length of this arrow represents its r value. Left, experimental condition of a generic monarch for ( a ) and ( b ). ( b ) Flight orientation of migrants with only a single antenna and housed in a 6-h-delayed LD cycle (light on between 1200 and 2400 hours). Migrants with both antennae intact were also tested in the 6-h-delayed LD cycle (green dots). Full size image Migrants with a single left antenna entrained to the 6-h-delayed LD cycle had an α of 351.7° ( n =6, r =0.86, P =0.006, Rayleigh's test) ( Fig. 1b , red solid circles), while those with a single right antenna housed under this same shifted LD cycle had a similar α of 6.14° ( n =6, r =0.99, P < 0.001, Raleigh's test) ( Fig. 1b , blue solid circles). There was no difference between the mean orientation of the migrants of both groups ( F 1, 10 =1.05, P =0.33, Watson–Williams F -test), and the combined α of both groups was 359.4° ( n =12, r =0.918, P < 0.0001, Rayleigh's test). Notably, there was a difference of 142° between the mean group orientation of the migrants housed in the 6-h-delayed LD cycle compared with the migrants housed in LD ( F 1, 22 =118.95, P <0.0001, Watson–Williams F -test). The clockwise direction and magnitude of the shift in the mean group orientation of the migrants housed under the 6-h-delayed LD cycle was consistent with that expected of a time-compensated sun compass that has been delayed by 6 h. The magnitude of the orientation difference between the LD and the 6-h-delayed LD groups was within the range of directions found in other studies examining the orientation of clock-delayed migrants [7] , [11] . Moreover, antenna removal had no effect on the group orientation direction manifested by the one-antenna migrants housed under the 6-h-delayed LD cycle, because control migrants with both antennae intact and housed under the same 6-h-delayed LD cycle had an α of 356.2° ( n =6, r =0.954, P <0.01, Rayleigh's test) ( Fig. 1b , green dots), which was not different from the mean orientation of migrants with either antenna (left: F 1, 10 =0.08, P =0.78; right: F 1, 10 =1.38, P =0.27, Watson–Williams F -test). These data demonstrate that a single antenna is sufficient to provide the circadian information necessary to calibrate the sun compass, allowing migrants to orient in a time-compensated way in the proper southwesterly direction. Furthermore, each of the two antennae is functionally equivalent for sun compass navigation. Conflicting antennal timing disrupts sun compass orientation We next asked whether there is asymmetry in the central integration of timing signals from each of the two antennae, as has been described for olfactory learning and memory in bees [8] , [9] , [10] . This was examined by determining whether the timing output from either antenna is equally sufficient to calibrate the sun compass in the presence of conflicting timing output from the other antenna. Migrants housed under LD had either the entire right or left antenna painted black and the other painted clear. The rationale for these treatments was that black paint would prevent light entrainment, thereby causing desynchronization among individual antennal clocks that would result in arrhythmic output from that antenna after several days [7] . To accelerate desynchronization of clocks among the black-painted antennae (see below), the black painting was performed throughout the light period of LD [12] , [13] . The clear paint, on the other hand, allowed for accurate light entrainment of the other antennae and served as a control for the painting process and the presence of paint [7] . We discovered that migrants with one black- and one clear-painted antennae had disoriented group flight orientation and that there was no apparent asymmetry in the central integration of the response ( Fig. 2a ). Migrants with either the right or left antenna painted black each oriented significantly, flying as strongly and consistently as migrants with unpainted antennae (see Methods ), but they were disoriented as a group (left black-painted: n =6, r =0.236, P =0.73, Rayleigh's test; right black-painted: n =6, r =0.382, P =0.43, Rayleigh's test; pooled: n =12, r =0.256, P =0.47, Rayleigh's test) ( Fig. 2a ). These data show that the timing output from a single light-entrained antenna (clear-painted) and the output from the paired antenna that has desynchronized antennal clocks (black-painted) are integrated in a way that overall disrupts proper flight orientation. Even though butterflies with conflicting antennal clocks lack appropriate time compensation to the changing sun angle, other aspects of the sun compass system such as the motivation and goal of directed flight remain intact, as they do in antennae-less migrants [7] . 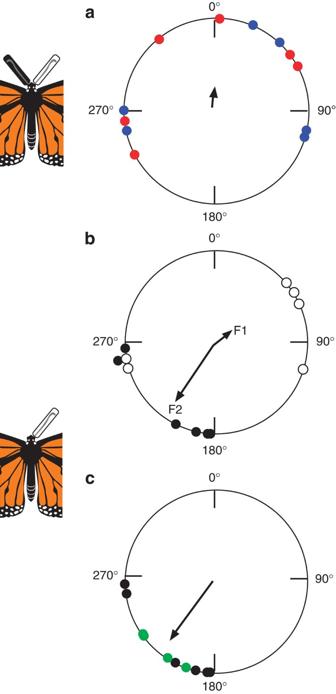Figure 2: Conflicting circadian timing between the two antennae disrupts sun compass orientation. (a) Flight orientation of migrants with a clear-painted and a black-painted antenna. Blue dots, left antenna painted black; red dots, right antenna painted black. Migrants were flown between 1300 and 1500 hours from 23 October to 20 November 2010. Left upper, experimental condition. (b) Flight orientation of migrants with painted antennae flown a second time after their black-painted antenna was removed. Open dots, first flight (F1 arrow) with clear- and black-painted antennae; black dots, second flight (F2) after black-painted antenna removed. Left lower, experimental condition for (b) and (c). (c) Combined flight orientation of migrants with only a clear-painted antenna. Green dots, first flight of migrants who had their black-painted antenna removed before their first flight trial; black dots, re-plotted from (b). Figure 2: Conflicting circadian timing between the two antennae disrupts sun compass orientation. ( a ) Flight orientation of migrants with a clear-painted and a black-painted antenna. Blue dots, left antenna painted black; red dots, right antenna painted black. Migrants were flown between 1300 and 1500 hours from 23 October to 20 November 2010. Left upper, experimental condition. ( b ) Flight orientation of migrants with painted antennae flown a second time after their black-painted antenna was removed. Open dots, first flight (F1 arrow) with clear- and black-painted antennae; black dots, second flight (F2) after black-painted antenna removed. Left lower, experimental condition for ( b ) and ( c ). ( c ) Combined flight orientation of migrants with only a clear-painted antenna. Green dots, first flight of migrants who had their black-painted antenna removed before their first flight trial; black dots, re-plotted from ( b ). Full size image Black antenna removal restores sun compass orientation We then asked whether we could restore oriented flight in the butterflies with conflicting antennal clocks by testing them a second time in the flight simulator, after removal of the black-painted antenna (thus removing the conflicting circadian information; see below). We indeed found that the re-flown migrants who previously had disoriented group flight direction when they possessed both black- and clear-painted antennae ( n =6, r =0.294, P =0.62, Rayleigh's test) now displayed oriented flight to the southwest once their black-painted antenna was removed ( α =214°, n =6, r =0.823, P =0.01, Rayleigh's test) ( Fig. 2c ). Similarly, we tested a second group of migrants also possessing one black- and one clear-painted antenna, but in which the black-painted antenna was removed before their virgin flight in the simulator. The flight of those migrants was also oriented southwest ( α =219°, n =4, r =0.969, P =0.01, Rayleigh's test), and the group orientation was similar to that of the second flight of the butterflies who had had the black-painted antenna removed ( F 1, 8 =0.07, P =0.80, Watson–Williams F -test). The combined α of both groups was 216° ( n =10, r =0.88, P <0.001, Rayleigh's test) ( Fig. 2c ). These results are consistent with the idea that the timing information from both antennae have a separate but similar role in calibrating the sun compass mechanism, and that the timing information from each is processed and integrated in the time-compensated sun compass circuit. Although it is unclear how and where this information is integrated, our data demonstrate that desynchronized timing output from one black antenna alters the processing of the timing output from a normally light-entrained antenna leading to disruption of the timing component of the sun compass mechanism. Molecular correlates of circadian timing To examine whether the timing of one antenna could directly influence the timing of the other, we evaluated molecular clock function in both black- and clear-painted antennae and brain from the same animals by assessing by quantitative real-time PCR (qPCR) the temporal patterns of messenger RNA expression of the period ( per ) and timeless ( tim ) genes at 3-h intervals over 24 h in LD. These genes were chosen because they exhibit robust mRNA cycling in the brain and unaltered antennae, and their oscillations provide reliable markers of the molecular clockwork [7] , [14] . Butterflies were studied in LD to match the conditions used for the flight orientation experiments. We found that the brains and clear-painted antenna of migrants had robust rhythmic expression patterns of per and tim in LD that were in phase with each other, with peak mRNA levels from Zeitgeber time (ZT) 12–18 and low levels from ZT 0–6, whereas the mean expression patterns of per and tim in the black-painted antennae were flat with little variation at each time point ( Fig. 3 ), consistent with desynchronized, dampened clocks. In a previous study from this laboratory, per and tim mRNA levels were found to be quite variable at each time point, and there was an apparent broadened mean daily oscillation, though it was not significantly rhythmic, consistent with comparably less desynchronization of clocks among the antennae of those animals [7] . However, in contrast to the current study in which black painting was performed throughout the light period of LD to accelerate desynchronization among antennae [12] , [13] , in the prior study black painting was performed within an hour prior of normal lights-off in LD, so that the clocks among those antennae began to free run at a similar ZT (ZT 11–12). Thus, the antennal molecular data from the current and previous study are consistent, even though in the current study the molecular rhythms were studied at 7 days after painting, compared with 11 days after painting in the prior study [7] . 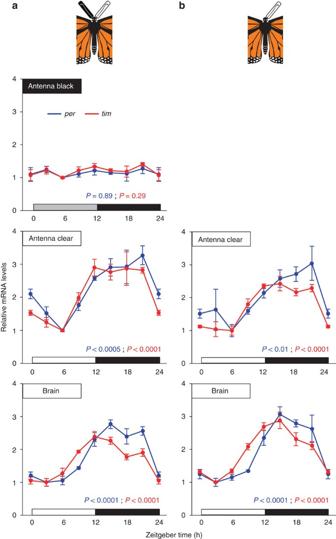Figure 3: Molecular correlates of circadian timing in the antennae and brain. (a) Antenna and brain profiles ofperandtimexpression in migrants with a clear- and black-painted antenna. Top, experimental condition for collections. Values are relative to the minimal level for each gene and are mean±s.e.m. of three antennae or three brains. Points at ZT 0 are re-plotted at ZT 24 to show the 24-h trend. Horizontal bars show the light cycle: open, lights on; grey, lights on in black-painted antenna; black, lights-off.P-values, one-way analysis of variance. (b) Antenna and brain profiles ofperandtimexpression in migrants in which the black-painted antenna was removed. Top, experimental condition for collections. Figure 3: Molecular correlates of circadian timing in the antennae and brain. ( a ) Antenna and brain profiles of per and tim expression in migrants with a clear- and black-painted antenna. Top, experimental condition for collections. Values are relative to the minimal level for each gene and are mean±s.e.m. of three antennae or three brains. Points at ZT 0 are re-plotted at ZT 24 to show the 24-h trend. Horizontal bars show the light cycle: open, lights on; grey, lights on in black-painted antenna; black, lights-off. P -values, one-way analysis of variance. ( b ) Antenna and brain profiles of per and tim expression in migrants in which the black-painted antenna was removed. Top, experimental condition for collections. Full size image These data show that although the clear-painted and black-painted antennae (from the same animals) each expressed different patterns of per and tim mRNA levels, neither antenna appeared to have a major influence on the pattern of gene expression of the other ( Fig. 3a ). Although we cannot rule out the possibility of weak coupling between the clocks of the paired antennae, the circadian clocks in an antenna did not appear to be substantially influenced by the altered timing of the paired antenna. Notably, robust rhythmic expression of per and tim in the brain occurred regardless of whether or not migrants were oriented as a group ( Fig. 3a,b ), again attesting to a negligible role of the brain clocks in timing sun compass orientation [7] . Molecular clocks throughout the length of the antenna We evaluated clock gene expression profiles in the two main regions of the antenna—the distal bulb and proximal flagellum shaft. This was done because the bulb is lightly pigmented at the tip compared with the more darkly pigmented flagellum ( Fig. 4a , inset), and it thus seemed possible that the light-entrained antennal clocks were localized to the bulb. qPCR was used to assess the temporal profiles of four clock-relevant genes. In addition to per and tim expression patterns, we also examined the temporal expression patterns of cryptochrome1 ( cry1 ) and cryptochrome2 ( cry2 ) mRNAs. cry1 encodes a blue-light photoreceptor that functions as a circadian photoreceptor in antennal clock cells [14] ; its expression pattern is not rhythmic [7] . cry2 encodes the major transcriptional repressor of the molecular clock feedback loop [14] , and its mRNA levels are rhythmically expressed in the antennae [7] . 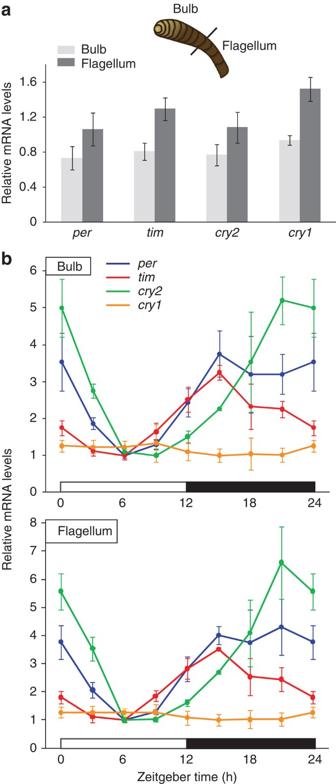Figure 4: Clock gene expression patterns do not vary between the antennal bulb and flagellum shaft. (a) mRNA expression in bulb and flagellum. Top inset is schematic of difference in cuticular pigmentation in bulb and flagellum; angled line, the dissection point to separate the two parts of the antenna. (b) Temporal profiles of clock gene expression in bulb (upper) and flagellum (lower) over the course of the day in LD. Values are relative to the minimal level for each gene and are the mean±s.e.m. of three animals. Statistical analysis performed using one-way analysis of variance.P-values for bulb:cry2, <0.0005;tim,<0.005;per, <0.05;cry1, >0.05. For flagellum:cry2, <0.0005;tim, <0.001;per, <0.01;cry1, >0.05. Figure 4: Clock gene expression patterns do not vary between the antennal bulb and flagellum shaft. ( a ) mRNA expression in bulb and flagellum. Top inset is schematic of difference in cuticular pigmentation in bulb and flagellum; angled line, the dissection point to separate the two parts of the antenna. ( b ) Temporal profiles of clock gene expression in bulb (upper) and flagellum (lower) over the course of the day in LD. Values are relative to the minimal level for each gene and are the mean±s.e.m. of three animals. Statistical analysis performed using one-way analysis of variance. P -values for bulb: cry2 , <0.0005; tim ,<0.005; per , <0.05; cry1 , >0.05. For flagellum: cry2 , <0.0005; tim , <0.001; per , <0.01; cry1 , >0.05. Full size image All four clock genes ( per , tim , cry1 and cry2 ) were expressed in both the antennal bulb and flagellum ( Fig. 4a ). In addition, the temporal expression patterns of the four clock genes were identical between the bulb and flagellum when studied in LD ( Fig. 4b ), and very similar to those previously reported in constant darkness [7] . Although these patterns were not examined in constant darkness, based on the prior whole-antenna studies [7] it would appear that light-entrained circadian clocks are distributed throughout the length of the monarch butterfly antenna. Cellular localization studies are needed to pinpoint where within antennal cellular architecture circadian clock cells actually reside and where they project. Our data solidify the critical role of the antennae in the navigational circuitry of monarch butterflies. Moreover, the results yield further insight into the mechanism of the time-compensated sun compass used by migratory monarchs. Specifically, we show that the necessary timing information from both antennae is likely integrated downstream from the clocks themselves. This downstream (output) integration is supported by the finding that the circadian clocks of one antenna do not appear to substantially alter the molecular timing of the other antenna, when the antennae are placed in conflict with one another. The two major neuronal outputs from the insect antennae include axons from mechanosensory cells that project to the antennal mechanosensory and motor centre in the central brain, and axons from olfactory neurons that innervate the antennal lobe [15] . Both outputs have been demonstrated in monarch butterflies [16] but whether either of these neural outputs contains the relevant timing information remains to be determined. No direct connection between the two antennal lobes exists to our knowledge. Alternatively, there may be a neuronal-independent output in which antennal clocks regulate the levels of a 'chronoactive' diffusible substance that communicates timing from the antennae to the sun compass complex in the brain. There is, in fact, precedent for clock-generated diffusible molecules regulating the circadian control of behaviours in both invertebrates [17] , [18] and vertebrates [19] , [20] . Regardless of the nature of the antennal clock output pathway, the timing information from either light-entrained antenna is sufficient to calibrate the sun compass, because removing one antenna does not alter proper group orientation to the southwest. Even though a single antenna is sufficient for proper sun compass orientation, the central integration of timing information from the light-entrained antenna is disrupted by the presence of a desynchronized antenna, leading to altered flight orientation and collectively disrupted group orientation ( Fig. 2a ), similar to the disorientation found when both antennae are missing [7] . Importantly, when the black-painted antenna is removed, the timing signals from the remaining light-entrained antenna can now be correctly used by the sun compass and normal orientation direction is restored ( Fig. 2b ). These results are consistent with the previous finding that when the clocks of both antennae are moderately desynchronized, the overall effect is persistent group orientation of improper direction, as the clocks are gradually free-running out of phase [7] . Thus, one antenna with fully desynchronized circadian clocks, along with its synchronized pair, is more disruptive for sun compass-mediated orientation than two co-existing, moderately desynchronized antennal clocks that remain somewhat in synchrony with each other. There is certainly a complex interplay between the outputs from the two antennae and resultant time compensation of the sun compass. Moreover, we do not yet know how the molecular oscillation in the antenna is ultimately translated into an output-timing signal. As previously proposed, brain circadian clocks appear to have little influence on the timing aspect of the sun compass system in the monarch butterfly [7] . Using the molecular oscillations of per and tim as molecular signatures of intact, unaltered clocks, the brain clock gene oscillations are virtually identical in oriented and disoriented butterflies. Although it is possible that clocks in the pars lateralis , the primary sites of brain clocks [14] , [21] , could be disrupted and their disrupted molecular oscillations missed in our whole-brain analyses, this seems unlikely given the profound effect of conflicting antennal timing on orientation behaviour and the tightly correlated temporal clock gene profiles from antennal clocks. Antennal clock control of sun compass orientation provides unusual evidence of peripheral clocks controlling a brain-mediated behaviour. The relationship between dual or physically separate clocks, and their coupling and regulation of brain-driven locomotor activity rhythms has been studied in hemimetabolous insects, such as the cockroach and cricket [22] , [23] , as well as in the sea slugs Bulla gouldiana [24] and Aplysia californica [25] , [26] . The dual clocks of the cockroach and cricket reside in the brain (optic lobes), are mutually coupled and are light-entrained by the eyes; a situation that is quite different from the butterfly antennal clocks. The closest paired-clock analogy to monarch antennal clocks are the eye clocks in Bulla and Aplysia . Similar to Aplysia eye clocks, the monarch antennal clocks may be weakly coupled. Both Aplisia eyes and monarch antennae represent paired organs with light-entrained circadian clocks whose timing is independent of each other but whose timing outputs are integrated to regulate a complex behaviour. However, the different behavioural outputs (locomotor activity rhythms versus time-compensated oriented flight) complicates brain-integration comparisons between the eye-mediated and antenna-mediated behaviours. Nonetheless, the properties of a dual timing system in the migratory monarch ensure accurate sun compass orientation even if parts of the antennae are lost during the long journey south. Animal rearing and housing Migratory monarch butterflies were captured by Fred Gagnon between 14 September and 1 October 2010, near Greenfield, MA (latitude 42°59′N, longitude 72°60′W). Migrants were housed indoors in glassine envelopes in either a Percival incubator that had its lighting regime set to coincide with prevailing fall light conditions (LD group), with lights on from 0600 to 1800 hours Eastern Standard Time (EST), or one in which the 12 h light:12 h dark lighting regime was delayed by 6 h (6-h-delayed LD group), with lights on from 1200 to 2400 hours. The temperature (21 °C) and humidity (70%) were controlled in the incubators. The butterflies were removed from their envelopes and fed a 25% honey solution every third day. Flight behaviour and analysis Monarchs of mixed sex were tethered for flight trials as described [4] and their flight behaviour was monitored using a flight simulator [27] . Flight simulator trials were conducted outdoors under sunny skies in Shrewsbury, MA (latitude 42°17′N, longitude 71°42′W), when the sun could be seen from the butterflies' position in the flight simulator. Flight studies were performed between 1300 and 1500 hours EST. Only butterflies flying continuously for a period of at least 5 min and presenting a directional flight path ( Z -scores >500) were considered for all analyses [11] . Of the 106 migrants tested in the flight simulator for these studies, 50 migrants (47%) flew continuously >5 min, consistent with prior results from this laboratory [7] , [11] . Of those 50 flying migrants, 46 flew directionally and were used for analysis; the 92% rate of individual directionality among fliers was consistent across experiments. For the migrants with black- and clear-painted antennae, 12 of the 13 that flew continuously for >5 min were directional. We determined the significance of orientation and the mean direction of the monarchs with circular statistics using the circular statistical package Oriana (Kovach Computing Services; http://www.kovcomp.com/ ). For single-antenna trials, we removed a single antenna (either the right or left) of a butterfly by clipping with a scissors at the base of the flagellum just above the pedicel [7] , and later monitored and assessed flight behaviour using a flight simulator. On average, the flight behaviour of these single-antenna monarchs was successfully assayed 11 days post removal of a single antenna (mean±s.e.m. : 10.83±0.98 days, range 6–23 days; n =24). For painted-antenna trials, we painted antennae from the tip to the base of the flagellum with either enamel-based clear paint (Model master clear top coat; Testors no. 2736) or black paint (Glossy black; Testors no. 1147) as previously described [7] . Our painting treatments consisted of one antenna painted black and the other painted clear. The black painting was performed throughout the light period of the LD cycle to help ensure more rapid desynchronization of the circadian clocks among black-painted antenna, as the migrant flight season was nearing its end; the completeness of painting was verified post-hoc under a dissecting scope. We tested monarchs in the flight simulator after at least 5 days after painting. The flight orientation of these monarchs was typically successfully assayed 8 days after an antenna was painted black (mean±s.e.m. : 7.67±0.72 days; range 5–14 days; n =12). We subsequently tested these monarchs a second time in flight simulator trials, in which we clipped the black-painted antenna and re-tested the monarchs with a clear-painted antenna alone. These butterflies were tested the second time after at least 4 days after removal of the black-painted antenna. The mean number of days that a monarch's flight orientation was successfully assayed was 11 days after the removal of the black-painted antenna (mean±s.e.m. : 10.5±1.77 days; range 4–16; n =6). We also performed control flight simulator trials in which monarchs had each antenna painted a different colour (that is, black or clear), but in which the black-painted antenna was removed before the first flight. The black-painted antenna of these monarchs was removed 6 days after painting. For this control group, we also tested butterflies after at least 2 days after the black-painted antenna was removed. The mean number of days that the orientation of these monarchs was assayed was 9 days after the removal of the black-painted antenna (mean±s.e.m. : 9±3.63 days; range 2–19 days; n =4). Tissue collection and qPCR Tissues were collected from the black- and clear-painted antennae and the brain of migrants at 7 days after painting, to correspond to the mean time the flight experiments were performed. For migrants in which the black antenna had been removed, the remaining clear-painted antenna and the brain were collected at 5 days after removal of the black-painted antenna, to correspond to the mean time the flight experiments were performed. The two bulbs and flagella of a pair of antennae from migrants were collected at ZT 12. Total RNA was extracted from the collected tissues using RNeasy Mini kit (Qiagen) and treated with RQ1 Dnase (Promega). Random hexamers (Promega) were used to prime reverse transcription with Superscript II (Invitrogen), according to the manufacturers' instructions. The quantifications of clock gene expression were performed by qPCR using TaqMan probes with an ABI Prism 7000 SDS (Applied Biosystems). PCR reactions were assembled by combining two master mixes. The monarch per , tim , cry1 , cry2 and control rp49 primers and probes were identical to those reported previously [14] . The efficiency of the amplification and detection by all primer and probesets were previously validated [14] . Individual reactions were used to quantify each RNA level in a given complementary DNA sample, and the average Ct from duplicated reactions within the same run was used for quantification. The data for each gene in a given tissue were normalized to rp49 as an internal control and normalized to the mean of one time point (for temporal profiling experiments) within a set for statistics. How to cite this article : Guerra P.A. et al . Discordant timing between antennae disrupts sun compass orientation in migratory monarch butterflies. Nat. Commun. 3:958 doi: 10.1038/ncomms1965 (2012).